BCR-signalling synergizes with TLR-signalling for induction of AID and immunoglobulin class-switching through the non-canonical NF-κB pathway By diversifying antibody biological effector functions, class switch DNA recombination has a central role in the maturation of the antibody response. Here we show that BCR-signalling synergizes with Toll-like receptor (TLR) signalling to induce class switch DNA recombination. BCR-signalling activates the non-canonical NF-κB pathway and enhances the TLR-dependent canonical NF-κB pathway, thereby inducing activation-induced cytidine deaminase (AID), which is critical for class switch DNA recombination. Escherichia coli lipopolysaccharide (LPS) triggers dual TLR4/BCR-signalling and induces hallmarks of BCR-signalling, including CD79a phosphorylation and Ca 2+ mobilization, and activates both the NF-κB pathways to induce AID and class switch DNA recombination in a PI(3)K p85α-dependent fashion. CD40-signalling activates the two NF-κB pathways to induce AID and class switch DNA recombination independent of BCR-signalling. Finally, dual BCR/TLR-engaging NP–lipopolysaccharide effectively elicits class-switched NP-specific IgG3 and IgG2b in mice. Thus, by integrating signals of the non-canonical and canonical NF-κB pathways, BCR and TLRs synergize to induce AID and T-cell-independent class switch DNA recombination. Innate immune receptors recognize conserved microbe-associated molecular patterns and have important roles in the early stages of the immune response [1] . Toll-like receptors (TLRs) are a family of conserved innate immune receptors highly expressed in macrophages, dendritic cells, epithelial cells and B cells [2] , [3] , [4] . Naïve B cells express a surface receptor for antigen (BCR) consisting of immunoglobulin (Ig)μ-chain (Igμ) and Igδ and react to antigens by making IgM and IgD antibodies (Abs). These are later diversified by somatic hypermutation (SHM) and class switch DNA recombination (CSR) [5] . SHM provides the structural substrate for antigen-mediated selection of higher affinity antibody mutants by introducing point-mutations with rare deletions or insertions into rearranged Ig variable regions. CSR replaces the Ig heavy chain (IgH) constant (C H ) region, for example, Cμ, with a downstream Cγ, Cα or C region, resulting in IgG, IgA or IgE antibodies with diverse biological effector functions [6] . Both SHM and CSR require activation-induced cytidine deaminase [6] (AID), which deaminates deoxycytidine, leading to the emergence of deoxyuracil [6] . This is not germane to DNA and is dealt with by elements of the DNA repair machinery, eventually leading to insertion of point-mutations in variable Ig regions for SHM and double-strand DNA breaks (DSBs) in switch (S) regions [6] , [7] , which lie 5′ of each of C H regions (except for Cδ), for CSR. CSR entails IgH locus germline I H -C H transcription, which is initiated by the I H promoter (Iμ, Iγ, Iα or I ) and proceeds through the upstream and downstream S and C H regions engaged in the CSR process, giving rise to germline Iμ-Cμ, Iγ-Cγ, Iα-Cα or I -C transcripts [6] . S regions contain a high density of 5′-AGCT-3′ repeats in their 'core' sequences. 5′-AGCT-3′ repeats recruit 14-3-3 adaptor proteins, which, in turn, target AID to S region DNA to generate DSBs [8] . CSR then proceeds through deletion of the intervening DNA and re-ligation of DSB free ends to form S–S junctions. The post-recombination sequences are transcribed, giving rise to post-recombination Iμ-Cγ, Iμ-Cα or Iμ-C transcripts and 'mature' V H DJ H -Cγ, V H DJ H -Cα or V H DJ H -C transcripts for the IgG, IgA or IgE H chain [6] . The efficiency of CSR critically depends on the level of AID [6] , [9] , which is under tight transcriptional regulation in a B-cell differentiation stage-specific fashion [10] , depending on HoxC4 (ref. 11 ), NF-κB (refs 11 , 12 ) and other transcription factors [12] , [13] , [14] . As shown by us [11] and others [12] , the NF-κB p52 subunit (a hallmark of the non-canonical NF-κB pathway [15] ) and p65 subunit (a hallmark of the canonical NF-κB pathway) bind to the AID gene ( AICDA/Aicda) promoter and upstream enhancers, respectively. AID and CSR are efficiently induced in T-dependent antibody responses by engagement of CD40 on B cells by surface CD154 (CD40 ligand) expressed on CD4 + T cells [15] and in the presence of appropriate cytokines (for example, IL-4, TGF-β or IFN-γ). However, IgG and IgA Abs can arise early in viral and bacterial infections before T-cell help becomes available [16] , indicating that CSR can also unfold in a T-cell-independent fashion. Accordingly, mice deficient in T cells or CD154/CD40 can generate class-switched specific Abs that are protective against some bacterial or viral infections [16] , [17] . In addition, class-switched Abs arise against bacterial or viral antigens that elicit weak or no T-cell responses (T-independent antigens), such as bacterial polysaccharides and lipolysaccharides (LPS) [18] , [19] . Further, polysaccharide-specific class-switched IgG Abs, which are critical for protection against infections by capsular bacteria [20] , are decreased in about half of patients deficient in the TLR-signalling molecule MyD88 or IRAK4 despite normal levels of total IgG/IgA Abs [21] . Finally, TLR ligands, for example, TLR4 ligand lipid A and TLR9 ligand CpG, can significantly boost specific antibody responses to proteinic (T-dependent) antigens [3] , [4] , [22] and, as such, are widely used as vaccine adjuvants. Despite the putative role of TLRs in class-switched antibody responses, only few studies exist on CSR induction by TLR ligands, including TLR3 ligand poly(I:C) [23] , TLR7 ligand 8-mercaptoguanosine or loxoribine [24] or CpG [25] . In these studies, TLR ligands alone triggered only marginal CSR, if at all [16] , [26] , suggesting that another B-cell-activating stimulus is required for TLR-dependent CSR induction. Indeed, engagement of selected surface B-cell molecules, such as CD38 (ref. 24 ), CD40 (ref. 25 ), CD180 (ref. 27 ), TACI (refs 23 , 25 , 28 ) and IL-10R (ref. 25 ), has been suggested to enhance TLR-dependent CSR. Likewise, TLR7- and TLR9-dependent CSR would be enhanced by BCR engagement [24] , [25] , [29] , albeit only marginally (1–4% B-cell switching) [24] , [25] . The mechanisms underlying a putative BCR enhancement of TLR-triggered CSR are unknown, in spite of findings suggesting an integration of BCR- and TLR-signalling for activation of NF-κB [30] and/or other transcription factors [31] , [32] , [33] , [34] . In contrast to other TLR ligands, LPS consists of a proper TLR-binding moiety (TLR4 ligand lipid A) and a repetitive polysaccharide moiety (O-antigen). This can elicit specific anti-polysaccharide antibody responses [19] through mobilization of O-antigen-binding B cells [35] . However, in spite of wide and empirical usage of LPS in mouse B cells, the mechanism underlying LPS-dependent CSR and its enhancement by BCR crosslinking [36] remain to be determined. Here we have tested the hypothesis that BCR-signalling synergizes with TLR-signalling for AID and CSR induction. We used a well-defined in vitro B-cell system to address the synergistic induction of CSR by BCR crosslinking [18] and the agonistic ligand of each one of the five TLRs highly expressed in B cells, that is, surface TLR1 and TLR2 (which form TLR1/2 heterodimer) and TLR4, and endosomal TLR7 and TLR9 (ref. 37 ). We further addressed the molecular mechanisms, underlying the synergy of BCR and TLR in inducing AID and CSR, by measuring activation of central components of the non-canonical and canonical NF-κB pathways and levels of AID expression, and by using B cells deficient in p85α ( p85α –/– ), the predominant class IA regulatory subunit of the PI(3)K lipid kinases that critically transduce BCR signals [38] . Finally, we analysed the unique properties of LPS in triggering dual BCR/TLR-signalling and, therefore, activating both the non-canonical and canonical NF-κB pathways for induction of AID and CSR. BCR synergizes with TLRs to induce CSR To test our hypothesis that BCR crosslinking provides a B-cell-specific signal enabling TLRs to induce CSR, we analysed CSR in B cells stimulated with agonistic ligands of surface TLR1/2 and TLR4 and endosomal TLR7 and TLR9. TLR1/2 ligand Pam 3 CSK 4 , TLR4 ligand lipid A, TLR7 ligand R-848 or TLR9 ligand CpG showed various B-cell mitogenic activities and, in the presence of appropriate cytokines, all induced only marginal CSR to IgG1, IgG2a, IgG3, IgA and IgE, even at a tenfold higher dose than that typically used ( Fig. 1 ; Supplementary Fig. S1 ). An agonistic anti-δ chain monoclonal Ab (mAb) conjugated to dextran (anti-δ mAb/dex), which crosslinks Igδ to trigger BCR-signalling and induces limited B-cell proliferation but no CSR [18] , synergized with these TLR ligands to induce CSR in a potent and dose-dependent fashion, as shown by analysis of surface (s)Ig ( Fig. 1 ; Supplementary Fig. S1 ), germline I H -C H , circle I H -Cμ, post-recombination Iμ-C H and mature V H DJ H -C H transcripts ( Fig. 2 ; Supplementary Fig. S2 ), and secreted Ig ( Supplementary Fig. S3 ). Anti-δ mAb/dex synergized with TLR ligands to induce CSR but not by enhancing B-cell proliferation, as it increased switched B cells at each cell division and over a tenfold range of CpG or LPS concentrations ( Fig. 1 and Fig. 2a,b ), and increased circle Iγ1-Cμ transcripts, an accurate parameter of ongoing CSR ( Fig. 2d ). Anti-δ mAb/dex did not further enhance CSR induced by membrane CD154 (mCD154) ( Fig. 1b ). Unlike anti-δ mAb/dex, BAFF or APRIL only moderately enhanced TLR-dependent CSR to IgG1, despite synergizing with anti-δ mAb/dex to induce CSR to IgA and, to a lesser extent, IgG1 ( Supplementary Fig. S4 ). BCR and TLR synergy in CSR induction was further emphasized by a decrease in anti-δ mAb/dex and CpG-induced CSR by chloroquine, an inhibitor of endosomal TLR maturation, and the negligible CSR induction by GpC, a weak TLR9 agonist [39] , and anti-δ mAb/dex ( Supplementary Fig. S5a ). Thus, BCR synergizes with TLR1/2, TLR4, TLR7 or TLR9 to induce efficient CSR; in the absence of BCR crosslinking, engagement of these TLRs alone results in only marginal CSR. 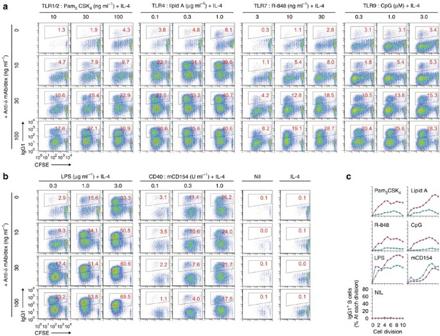Figure 1: BCR crosslinking enables TLRs to induce efficient CSR. (a) Proportions of surface IgG1+(sIgG1+) B cells after stimulation of CFSE-labelled sIgδ+B cells with TLR1/2 ligand Pam3CSK4, TLR4 ligand lipid A, TLR7 ligand R-848 or TLR9 ligand CpG at indicated doses, in the absence or presence of anti-δ mAb/dex at indicated doses, plus IL-4 (3 ng ml−1). (b) Proportions of sIgG1+B cells at each cell division after stimulation of sIgδ+B cells with LPS or mCD154 at indicated doses, in the absence or presence of anti-δ mAb/dex (100 ng ml−1), plus IL-4 (3 ng ml−1). (c) Proportions of sIgG1+B cells within each B cell division after stimulation of CFSE-labelled sIgδ+B cells with Pam3CSK4(100 ng ml−1), lipid A (1 μg ml−1), R-848 (30 ng ml−1), CpG (1 μM), LPS (3 μg ml−1) or mCD154 (1 U ml−1), in the absence (teal) or presence (plum) of anti-δ mAb/dex (100 ng ml−1), plus IL-4 (3 ng ml−1). Data are representative of four independent experiments. Figure 1: BCR crosslinking enables TLRs to induce efficient CSR. ( a ) Proportions of surface IgG1 + (sIgG1 + ) B cells after stimulation of CFSE-labelled sIgδ + B cells with TLR1/2 ligand Pam 3 CSK 4 , TLR4 ligand lipid A, TLR7 ligand R-848 or TLR9 ligand CpG at indicated doses, in the absence or presence of anti-δ mAb/dex at indicated doses, plus IL-4 (3 ng ml −1 ). ( b ) Proportions of sIgG1 + B cells at each cell division after stimulation of sIgδ + B cells with LPS or mCD154 at indicated doses, in the absence or presence of anti-δ mAb/dex (100 ng ml −1 ), plus IL-4 (3 ng ml −1 ). ( c ) Proportions of sIgG1 + B cells within each B cell division after stimulation of CFSE-labelled sIgδ + B cells with Pam 3 CSK 4 (100 ng ml −1 ), lipid A (1 μg ml −1 ), R-848 (30 ng ml −1 ), CpG (1 μ M ), LPS (3 μg ml −1 ) or mCD154 (1 U ml −1 ), in the absence (teal) or presence (plum) of anti-δ mAb/dex (100 ng ml −1 ), plus IL-4 (3 ng ml −1 ). Data are representative of four independent experiments. 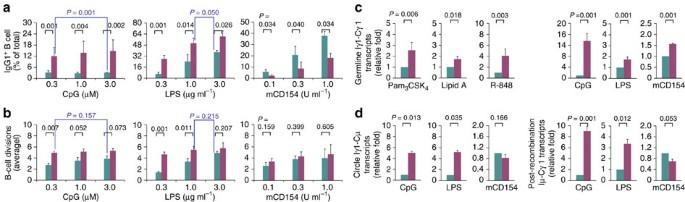Figure 2: BCR crosslinking potentiates TLR-dependent CSR in a proliferation-independent fashion. (a,b) Proportions of sIgG1+B cells (a) and average B-cell divisions (b) after stimulation of CFSE-labelled sIgδ+B cells with CpG, LPS or mCD154, at indicated doses, plus IL-4 (3 ng ml−1) in the absence (teal) or presence (plum) of anti-δ mAb/dex (100 ng ml−1) (mean and s.e.m. of data from four independent experiments). Also depicted (blue brackets) are higher CSR rates in B cells stimulated with low dosages of CpG or LPS in the presence of anti-δ mAb/dex than in B cells stimulated with high dosages of CpG or LPS in the absence of anti-δ mAb/dex (despite comparable proliferation).Pvalues:t-test. (c) Levels of germline Iγ1-Cγ1 transcripts in B cells stimulated for 48 h with TLR ligand Pam3CSK4(100 ng ml−1), lipid A (1 μg ml−1), R-848 (30 ng ml−1), CpG (1 μM), LPS (3 μg ml−1) or mCD154 (1 U ml−1), plus IL-4 (3 ng ml−1) in the absence (teal) or presence (plum) of anti-δ mAb/dex. Data were normalized to the level ofCd79band are depicted as the ratio to the expression levels in B cells stimulated in the absence of anti-δ mAb/dex (mean and s.e.m. of data from three independent experiments;Pvalues:t-test). (d) Levels of circle Iγ1-Cμ transcripts and post-recombination Iμ-Cγ1 transcripts in B cells stimulated with CpG (1 μM), LPS (3 μg ml−1) or mCD154 (1 U ml−1) plus IL-4 (3 ng ml−1) in the absence (teal) or presence (plum) of anti-δ mAb/dex for 48 h. Data were normalized to the level ofCd79band are depicted as the ratio to the expression levels in B cells stimulated in the absence of anti-δ mAb/dex (mean and s.e.m. of data from three independent experiments;Pvalues:t-test). Full size image Figure 2: BCR crosslinking potentiates TLR-dependent CSR in a proliferation-independent fashion. ( a,b ) Proportions of sIgG1 + B cells ( a ) and average B-cell divisions ( b ) after stimulation of CFSE-labelled sIgδ + B cells with CpG, LPS or mCD154, at indicated doses, plus IL-4 (3 ng ml −1 ) in the absence (teal) or presence (plum) of anti-δ mAb/dex (100 ng ml −1 ) (mean and s.e.m. of data from four independent experiments). Also depicted (blue brackets) are higher CSR rates in B cells stimulated with low dosages of CpG or LPS in the presence of anti-δ mAb/dex than in B cells stimulated with high dosages of CpG or LPS in the absence of anti-δ mAb/dex (despite comparable proliferation). P values: t -test. ( c ) Levels of germline Iγ1-Cγ1 transcripts in B cells stimulated for 48 h with TLR ligand Pam 3 CSK 4 (100 ng ml −1 ), lipid A (1 μg ml −1 ), R-848 (30 ng ml −1 ), CpG (1 μ M ), LPS (3 μg ml −1 ) or mCD154 (1 U ml −1 ), plus IL-4 (3 ng ml −1 ) in the absence (teal) or presence (plum) of anti-δ mAb/dex. Data were normalized to the level of Cd79b and are depicted as the ratio to the expression levels in B cells stimulated in the absence of anti-δ mAb/dex (mean and s.e.m. of data from three independent experiments; P values: t -test). ( d ) Levels of circle Iγ1-Cμ transcripts and post-recombination Iμ-Cγ1 transcripts in B cells stimulated with CpG (1 μ M ), LPS (3 μg ml −1 ) or mCD154 (1 U ml −1 ) plus IL-4 (3 ng ml −1 ) in the absence (teal) or presence (plum) of anti-δ mAb/dex for 48 h. Data were normalized to the level of Cd79b and are depicted as the ratio to the expression levels in B cells stimulated in the absence of anti-δ mAb/dex (mean and s.e.m. of data from three independent experiments; P values: t -test). Full size image LPS induces BCR-signalling for CSR LPS, unlike its lipid A moiety, induced AID and CSR to all Ig isotypes ( Fig. 1b ; Supplementary Fig. S1 and ref. 6 ), suggesting LPS fulfills the requirement of dual BCR/TLR-signalling by engaging TLR4 through the lipid A moiety and BCR through the polysaccharidic moiety, respectively. In the normal B-cell repertoire, many B cells express BCRs that bind with variable affinities to repetitive polysaccharides [35] , which include the polysaccharidic moiety of LPS. Indeed, CD79a Tyr182, one of the two ITAM Tyr residues, which, on phosphorylation, transduce BCR-signalling [29] , was phosphorylated in B cells stimulated with anti-δ mAb/dex or anti-μ F(ab′) 2 or LPS (within 3 h, and more within 24 h), but not lipid A ( Fig. 3a ). In addition, unlike anti-μ F(ab′) 2 , which induced a rapid increase of free cytosolic Ca 2+ ions ([Ca 2+ ] cytosol ), anti-δ mAb/dex induced a slower, but continuous increase in [Ca 2+ ] cytosol ( Fig. 3b ). As sustained extracellular Ca 2+ entry is required upon BCR engagement for activation of Ca 2+ -dependent signalling pathways, we pretreated B cells with LPS, anti-δ mAb/dex, lipid A or mCD154, followed by labelling with Ca 2+ indicator dyes and then probing for Ca 2+ mobilization in response to anti-μ F(ab′) 2 . B cells, pretreated for 16 h with LPS or anti-δ mAb/dex, showed only a transient Ca 2+ flux on further stimulation with anti-μ F(ab′) 2 , likely resulting from Ca 2+ release from ER stores only and without the sustained entry of Ca 2+ from the plasma membrane [40] , as it occurred in B cells that were pretreated with lipid A or mCD154 ( Fig. 3c ). This suggests that LPS or anti-δ mAb/dex likely triggered sustained Ca 2+ elevation before the B cells were rendered refractory to extra Ca 2+ entry. Finally, LPS-induced CSR could be further increased by anti-δ mAb/dex ( Fig. 1b ; Supplementary Fig. S1 ), which inhibited LPS-induced plasmacytoid differentiation ( Supplementary Fig. S5b ), resulting in virtually no increase in secreted IgG1 or IgE ( Supplementary Fig. S3 ). These experiments show that LPS triggers dual BCR/TLR-signalling by engaging TLR4 through lipid A and by inducing CD79a Tyr phosphorylation and Ca 2+ mobilization (hallmark BCR-signalling events). 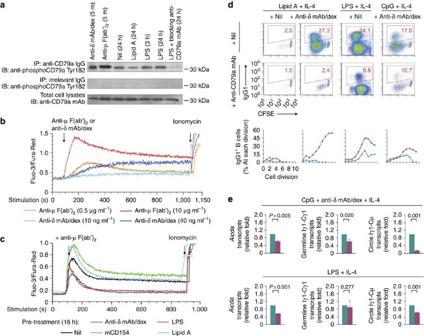Figure 3: LPS induces BCR-signalling, and blocking of CD79a inhibits CSR induced by dual BCR/TLR engagement or LPS. (a) CD79a phosphorylation in B cells stimulated with anti-δ mAb/dex (100 ng ml−1) for 5 m, anti-μ F(ab′)2(5 μg ml−1) for 5 m, nil, lipid A (1 μg ml−1) for 24 h, LPS (3 μg ml−1) for 3 h or 24 h, or LPS (3 μg ml−1) plus blocking anti-CD79a mAb for 24 h. (b) Ca2+mobilization in B cells stimulated with anti-μ F(ab′)2or anti-δ mAb/dex at indicated doses for a short period (less than 30 m). (c) Anti-μ F(ab′)2–triggered Ca2+mobilization in B cells pretreated with nil, anti-δ mAb/dex (100 ng ml−1), LPS (3 μg ml−1), lipid A (1 μg ml−1) or mCD154 (1 U ml−1) for 16 h (elevated [Ca2+]cytosolwould reduce the amplitude of the Ca2+flux and subsequent steady-state Ca2+levels induced by newly applied anti-μ F(ab′)2). Data are representative of three independent experiments. (d) Proportions of sIgG1+B cells after stimulation of CFSE-labelled sIgδ+B cells with lipid A in the absence (teal) or presence (plum) of anti-δ mAb/dex (100 ng ml−1), LPS (3 μg ml−1), or CpG (1 μM) in the presence of anti-δ mAb/dex, plus IL-4 (3 ng ml−1) and treated with nil or blocking anti-CD79a mAb (1 μg ml−1) (top panels). Also depicted are proportions of B cells at each cell division that were IgG1+(bottom panels). (e) Levels ofAicda, germline Iγ1-Cγ1 and circle Iγ1-Cμ transcripts in B cells stimulated with CpG (1 μM) and anti-δ mAb/dex (100 ng ml−1), or LPS (3 μg ml−1), in the absence (teal) or presence (plum) of blocking anti-CD79a mAb (1 μg ml−1) (all with 3 ng ml−1of IL-4). Data were normalized to the level ofCd79band are depicted as the ratio to the expression levels in B cells not treated with anti-CD79a mAb (mean and s.e.m. of data from three independent experiments;Pvalues:t-test). Figure 3: LPS induces BCR-signalling, and blocking of CD79a inhibits CSR induced by dual BCR/TLR engagement or LPS. ( a ) CD79a phosphorylation in B cells stimulated with anti-δ mAb/dex (100 ng ml −1 ) for 5 m, anti-μ F(ab′) 2 (5 μg ml −1 ) for 5 m, nil, lipid A (1 μg ml −1 ) for 24 h, LPS (3 μg ml −1 ) for 3 h or 24 h, or LPS (3 μg ml −1 ) plus blocking anti-CD79a mAb for 24 h. ( b ) Ca 2+ mobilization in B cells stimulated with anti-μ F(ab′) 2 or anti-δ mAb/dex at indicated doses for a short period (less than 30 m). ( c ) Anti-μ F(ab′) 2 –triggered Ca 2+ mobilization in B cells pretreated with nil, anti-δ mAb/dex (100 ng ml −1 ), LPS (3 μg ml −1 ), lipid A (1 μg ml −1 ) or mCD154 (1 U ml −1 ) for 16 h (elevated [Ca 2+ ] cytosol would reduce the amplitude of the Ca 2+ flux and subsequent steady-state Ca 2+ levels induced by newly applied anti-μ F(ab′) 2 ). Data are representative of three independent experiments. ( d ) Proportions of sIgG1 + B cells after stimulation of CFSE-labelled sIgδ + B cells with lipid A in the absence (teal) or presence (plum) of anti-δ mAb/dex (100 ng ml −1 ), LPS (3 μg ml −1 ), or CpG (1 μ M ) in the presence of anti-δ mAb/dex, plus IL-4 (3 ng ml −1 ) and treated with nil or blocking anti-CD79a mAb (1 μg ml −1 ) (top panels). Also depicted are proportions of B cells at each cell division that were IgG1 + (bottom panels). ( e ) Levels of Aicda , germline Iγ1-Cγ1 and circle Iγ1-Cμ transcripts in B cells stimulated with CpG (1 μ M ) and anti-δ mAb/dex (100 ng ml −1 ), or LPS (3 μg ml −1 ), in the absence (teal) or presence (plum) of blocking anti-CD79a mAb (1 μg ml −1 ) (all with 3 ng ml −1 of IL-4). Data were normalized to the level of Cd79b and are depicted as the ratio to the expression levels in B cells not treated with anti-CD79a mAb (mean and s.e.m. of data from three independent experiments; P values: t -test). Full size image BCR-signalling increases TLR-dependent Aicda expression Consistent with its potentiation of TLR-dependent CSR, anti-δ mAb/dex, which alone did not induce AID expression, significantly increased Aicda transcripts induced by TLR ligand Pam 3 CSK 4 , lipid A, R-848 or CpG (in the presence of IL-4), resulting in Aicda levels (peaking at 60 h) comparable to those induced by LPS ( Fig. 4a,b ). Anti-δ mAb/dex decreased mCD154 and IL-4-induced AID expression, consistent with its reduction of CD40-dependent CSR to IgG1 ( Fig. 1b ). Anti-δ mAb/dex enhanced, to variable extents, germline Iγ1-Cγ1 transcription induced by IL-4 or IL-4 and TLR ligands (peaking as early as at 12 h) or mCD154. It also upregulated B-cell expression of PNA-binding glycoproteins, which are markers of germinal centre B cells, as induced by CpG, but not CD40—high levels of PNA-binding glycoproteins induced by LPS were not further increased by anti-δ mAb/dex ( Fig. 4c ; Supplementary Fig. S5c ). Anti-δ mAb/dex downregulated Blimp1 and CD138 expression ( Fig. 4a,d ), consistent with inhibition of plasmacytoid differentiation by BCR-signalling [41] . To further confirm that BCR-signalling increases TLR-dependent Aicda expression and CSR, we blocked BCR-signalling with an anti-CD79a mAb, which inhibited LPS-induced CD79a phosphorylation ( Fig. 3a ). This blocking anti-CD79a mAb significantly reduced the levels of Aicda transcripts and inhibited CSR to IgG1, resulting in decreased levels of sIgG1 and circle Iγ1-Cμ transcripts, as induced by the BCR/TLR dual engagement or LPS ( Fig. 3d,e ). Finally, that BCR signalling enabled TLR-dependent CSR by upregulating AID expression was demonstrated by the ability of exogenous AID to substitute anti-δ mAb/dex in TLR9-dependent CSR ( Fig. 4e,f ). Thus, BCR-signalling enables TLR-dependent induction of efficient CSR by enhancing TLR-dependent AID induction. It also enhances TLR-dependent expression of PNA-binding glycoproteins and suppresses plasmacytoid differentiation. 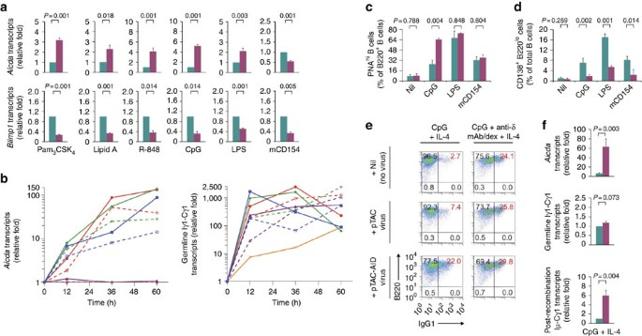Figure 4: BCR crosslinking increases TLR-dependent AID expression. (a)AicdaandBlimp1transcripts in B cells stimulated for 48 h with Pam3CSK4(100 ng ml−1), lipid A (1 μg ml−1), R-848 (30 ng ml−1), CpG (1 μM), LPS (3 μg ml−1) or mCD154 (1 U ml−1) plus IL-4 (3 ng ml−1) in the absence (teal) or presence (plum) of anti-δ mAb/dex (100 ng ml−1). Data were normalized to the level ofCd79band are depicted as the ratio to the expression levels in B cells stimulated in the absence of anti-δ mAb/dex (mean and s.e.m. of data from three independent experiments;Pvalues:t-test). (b) Kinetics of induction of AID expression and germline Iγ1-Cγ1 transcription by anti-δ mAb/dex alone (100 ng ml−1, orange), IL-4 (3 ng ml−1, purple triangles) or lipid A (1 μg ml−1, green diamonds), CpG (1 μM, blue squares) or LPS (3 μg ml−1, red circles) plus IL-4 in the absence (open symbols) or presence (filled symbols) of anti-δ mAb/dex. Levels ofAicdaand germline Iγ1-Cγ1 transcripts were normalized to the level ofCd79band are depicted as the ratio to the expression levels in unstimulated sIgδ+B cells (0 h, set as 1). Anti-δ mAb/dex alone induced only low levels of germline Iγ1-Cγ1 transcription. Data are representative of three independent experiments. (c) Proportions of PNAhi(B220+) B cells after stimulation of sIgδ+B cells with nil, anti-δ mAb/dex (100 ng ml−1), or CpG (1 μM), LPS (3 μg ml−1) or mCD154 (1 U ml−1) in the absence (teal) or presence (plum) of anti-δ mAb/dex (all in the presence of 3 ng ml−1of IL-4, mean and s.e.m. of data from three independent experiments,Pvalues:t-test). (d) Proportions of CD138+(Syndecan-1+) B220loplasmacytoid cells/plasmacytes after stimulation of sIgδ+B cells with nil, anti-δ mAb/dex (100 ng ml−1), or CpG (1 μM), LPS (3 μg ml−1) or mCD154 (1 U ml−1) in the absence (teal) or presence (plum) of anti-δ mAb/dex (all in the presence of 3 ng ml−1of IL-4, mean and s.e.m. of data from three independent experiments,Pvalues:t-test). (e) Potentiation of TLR9-dependent CSR to IgG1 by exogenous AID. Proportions of sIgG1+(B220+) B cells after sIgδ+B cells were transduced with pTAC or pTAC–AID retrovirus (CD25+) and stimulated with CpG (1 μM), or CpG and anti-δ mAb/dex (100 ng ml−1), plus IL-4 (3 ng ml−1). (f) Levels ofAicda, germline Iγ1-Cγ1 and post-recombination Iμ-Cγ1 transcripts in B cells transduced with pTAC (teal) or pTAC–AID (plum) retrovirus and stimulated with CpG (1 μM) plus IL-4 (3 ng ml−1). Data were normalized to the level ofCd79band are depicted as the ratio to the expression levels in the B cells transduced with pTAC virus (mean and s.d. of triplicate samples,Pvalues:t-test). Figure 4: BCR crosslinking increases TLR-dependent AID expression. ( a ) Aicda and Blimp1 transcripts in B cells stimulated for 48 h with Pam 3 CSK 4 (100 ng ml −1 ), lipid A (1 μg ml −1 ), R-848 (30 ng ml −1 ), CpG (1 μ M ), LPS (3 μg ml −1 ) or mCD154 (1 U ml −1 ) plus IL-4 (3 ng ml −1 ) in the absence (teal) or presence (plum) of anti-δ mAb/dex (100 ng ml −1 ). Data were normalized to the level of Cd79b and are depicted as the ratio to the expression levels in B cells stimulated in the absence of anti-δ mAb/dex (mean and s.e.m. of data from three independent experiments; P values: t -test). ( b ) Kinetics of induction of AID expression and germline Iγ1-Cγ1 transcription by anti-δ mAb/dex alone (100 ng ml −1 , orange), IL-4 (3 ng ml −1 , purple triangles) or lipid A (1 μg ml −1 , green diamonds), CpG (1 μ M , blue squares) or LPS (3 μg ml −1 , red circles) plus IL-4 in the absence (open symbols) or presence (filled symbols) of anti-δ mAb/dex. Levels of Aicda and germline Iγ1-Cγ1 transcripts were normalized to the level of Cd79b and are depicted as the ratio to the expression levels in unstimulated sIgδ + B cells (0 h, set as 1). Anti-δ mAb/dex alone induced only low levels of germline Iγ1-Cγ1 transcription. Data are representative of three independent experiments. ( c ) Proportions of PNA hi (B220 + ) B cells after stimulation of sIgδ + B cells with nil, anti-δ mAb/dex (100 ng ml −1 ), or CpG (1 μ M ), LPS (3 μg ml −1 ) or mCD154 (1 U ml −1 ) in the absence (teal) or presence (plum) of anti-δ mAb/dex (all in the presence of 3 ng ml −1 of IL-4, mean and s.e.m. of data from three independent experiments, P values: t -test). ( d ) Proportions of CD138 + (Syndecan-1 + ) B220 lo plasmacytoid cells/plasmacytes after stimulation of sIgδ + B cells with nil, anti-δ mAb/dex (100 ng ml −1 ), or CpG (1 μ M ), LPS (3 μg ml −1 ) or mCD154 (1 U ml −1 ) in the absence (teal) or presence (plum) of anti-δ mAb/dex (all in the presence of 3 ng ml −1 of IL-4, mean and s.e.m. of data from three independent experiments, P values: t -test). ( e ) Potentiation of TLR9-dependent CSR to IgG1 by exogenous AID. Proportions of sIgG1 + (B220 + ) B cells after sIgδ + B cells were transduced with pTAC or pTAC–AID retrovirus (CD25 + ) and stimulated with CpG (1 μ M ), or CpG and anti-δ mAb/dex (100 ng ml −1 ), plus IL-4 (3 ng ml −1 ). ( f ) Levels of Aicda , germline Iγ1-Cγ1 and post-recombination Iμ-Cγ1 transcripts in B cells transduced with pTAC (teal) or pTAC–AID (plum) retrovirus and stimulated with CpG (1 μ M ) plus IL-4 (3 ng ml −1 ). Data were normalized to the level of Cd79b and are depicted as the ratio to the expression levels in the B cells transduced with pTAC virus (mean and s.d. of triplicate samples, P values: t -test). Full size image BCR and TLR activate both NF-κB pathways for AID induction We next addressed the mechanisms underlying the synergy of BCR and TLRs in inducing AID expression, which is regulated by the HoxC4 and NF-κB transcription factors [11] , [12] . Anti-δ mAb/dex did not enhance TLR-induced expression of HoxC4, prompting us to hypothesize that BCR and TLRs synergize to induce AID by activating both the canonical NF-κB (p65) and non-canonical NF-κB (p52) pathways, as CD40 does [15] . To test this hypothesis, we tracked the kinetics of IκBα phosphorylation at Ser32 and p65 phosphorylation at Ser536 (canonical) and expression of p100, the precursor of p52, and processing of p100 to p52 (non-canonical) in B cells stimulated with TLR ligands, anti-δ mAb/dex, or both (all in the presence of IL-4). Consistent with the findings that TLRs activate the canonical NF-κB pathway [2] , CpG or lipid A induced IκBα and p65 phosphorylation that did not peak until 40 m after stimulation. These phosphorylation events were accelerated and enhanced by anti-δ mAb/dex, as were IκBα and p65 phosphorylation induced by LPS, but not CD40 ( Fig. 5 ; Supplementary Fig. S6 ). Anti-δ mAb/dex alone, however, did not activate appreciable p65 phosphorylation ( Supplementary Fig. S6a ). Rather, it increased the level of both p52 and p100 within 24–48 h, the time frame of AID induction, as mCD154 did ( Fig. 6a ; Supplementary Fig. S7a ). Like anti-δ mAb/dex, LPS increased the levels of p100 and p52. Lipid A, or CpG, mainly increased p100, thereby providing more substrate for anti-δ mAb/dex-processing to p52 ( Fig. 6a ). Thus, BCR and TLRs each activates only one NF-κB pathway (non-canonical and canonical, respectively), but reciprocally enhance the main pathway of activation by the other receptor, thereby synergizing in inducing AID expression, as mediated by both NF-κB pathways. 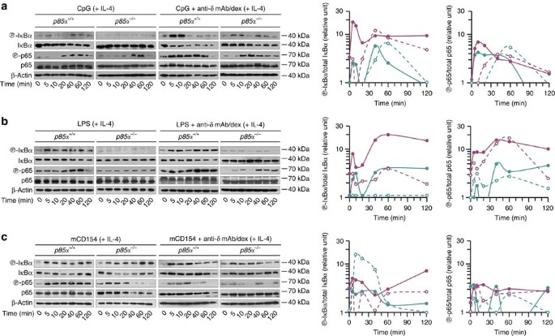Figure 5: BCR crosslinking enhances the TLR-dependent canonical NF-κB pathway in a p85α-dependent fashion. (a–c) Levels of phosphorylated IκBα, total IκBα, phosphorylated p65, total p65 and β-actin inp85α+/+(plum) andp85α–/–(teal) B cells stimulated with CpG (1 μM), LPS (3 μg ml−1) or mCD154 (1 U ml−1) plus IL-4 (3 ng ml−1) in the absence (open symbols) or presence (filled symbols) of anti-δ mAb/dex (100 ng ml−1) (left panels; the IκBα degradation and subsequent re-synthesis led to more than one peak of IκBα phosphorylation). Levels of phosphorylated IκBα and p65 were normalized to the level of total IκBα and p65, respectively, and data are depicted as the ratio to the expression levels inp85α–/–B cells before stimulation (0 m, set as 1; right panels). Inp85α–/–B cells, p65 phosphorylation induced by CpG or mCD154 was not impaired despite changes in IκBα phosphorylation, that is, decrease following stimulation with CpG and increase following stimulation with mCD154. Data are representative of three independent experiments. Figure 5: BCR crosslinking enhances the TLR-dependent canonical NF-κB pathway in a p85α-dependent fashion. ( a–c ) Levels of phosphorylated IκBα, total IκBα, phosphorylated p65, total p65 and β-actin in p85α +/+ (plum) and p85α –/– (teal) B cells stimulated with CpG (1 μ M ), LPS (3 μg ml −1 ) or mCD154 (1 U ml −1 ) plus IL-4 (3 ng ml −1 ) in the absence (open symbols) or presence (filled symbols) of anti-δ mAb/dex (100 ng ml −1 ) (left panels; the IκBα degradation and subsequent re-synthesis led to more than one peak of IκBα phosphorylation). Levels of phosphorylated IκBα and p65 were normalized to the level of total IκBα and p65, respectively, and data are depicted as the ratio to the expression levels in p85α –/– B cells before stimulation (0 m, set as 1; right panels). In p85α –/– B cells, p65 phosphorylation induced by CpG or mCD154 was not impaired despite changes in IκBα phosphorylation, that is, decrease following stimulation with CpG and increase following stimulation with mCD154. Data are representative of three independent experiments. 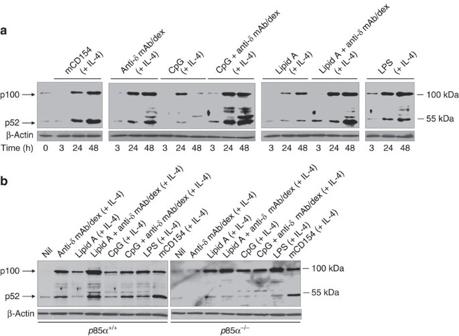Figure 6: BCR crosslinking activates the non-canonical NF-κB pathway in a p85α-dependent fashion. (a) Induction of p52 and p100 in B cells stimulated with anti-δ mAb/dex (100 ng ml−1), lipid A (1 μg ml−1) or CpG (1 μM) in the absence or presence of anti-δ mAb/dex, LPS (3 μg ml−1) or mCD154 (1 U ml−1) (all in the presence of 3 ng ml−1of IL-4) for 0, 3, 24 and 48 h. (b) Levels of p52, p100 and β-actin inp85α+/+andp85α–/–B cells stimulated with anti-δ mAb/dex (100 ng ml−1), lipid A (1 μg ml−1) or CpG (1 μM) in the absence or presence of anti-δ mAb/dex, LPS (3 μg ml−1) or mCD154 (1 U ml−1) (all in the presence of 3 ng ml−1of IL-4) for 48. Data are representative of three independent experiments. Full size image Figure 6: BCR crosslinking activates the non-canonical NF-κB pathway in a p85α-dependent fashion. ( a ) Induction of p52 and p100 in B cells stimulated with anti-δ mAb/dex (100 ng ml −1 ), lipid A (1 μg ml −1 ) or CpG (1 μ M ) in the absence or presence of anti-δ mAb/dex, LPS (3 μg ml −1 ) or mCD154 (1 U ml −1 ) (all in the presence of 3 ng ml −1 of IL-4) for 0, 3, 24 and 48 h. ( b ) Levels of p52, p100 and β-actin in p85α +/+ and p85α –/– B cells stimulated with anti-δ mAb/dex (100 ng ml −1 ), lipid A (1 μg ml −1 ) or CpG (1 μ M ) in the absence or presence of anti-δ mAb/dex, LPS (3 μg ml −1 ) or mCD154 (1 U ml −1 ) (all in the presence of 3 ng ml −1 of IL-4) for 48. Data are representative of three independent experiments. Full size image NF-κB activation by BCR/TLR engagement requires PI(3)K As PI(3)K transduces BCR-signalling [38] , we next used p85α –/– B cells to explore the impact of impaired BCR-signalling on activation of the two NF-κB pathways and, therefore, TLR-dependent AID expression and CSR. Mature p85α –/– B cells expressed normal sIgδ levels [38] and, on stimulation with mCD154, showed normal proliferation and slightly higher levels of CSR than their p85α +/+ counterparts, likely owing to impairment in the tonic BCR-signalling that would have decreased CD40-dependent CSR ( Fig. 7 ). In addition, anti-δ mAb/dex did not affect CD40-dependent CSR in p85α –/– B cells ( Fig. 7; Supplementary Fig. S8 ). On stimulation with Pam 3 CSK 4 , lipid A, R-848 or CpG, p85α –/– B cells underwent limited CSR, as their p85α +/+ counterparts did. This and the comparable proliferation of TLR ligand-stimulated p85α –/– and p85α +/+ B cells demonstrated that p85α was not instrumental in transducing TLR-signalling in B cells. Anti-δ mAb/dex potentiation of TLR-dependent CSR, however, was impaired in p85α –/– B cells, even after normalization to cell division—the residual CSR likely resulted from BCR-signalling mediated by minor PI(3)K regulatory subunits [38] ( Fig. 7a,b; Supplementary Fig. S8 ). LPS-induced CSR was also impaired in p85α –/– B cells, consistent with an important role of BCR-signalling in this process. The decrease in dual BCR/TLR engagement or LPS-induced CSR to IgG1 in p85α –/– B cells was associated with significantly reduced Aicda , germline (Iγ1-Cγ1), circle (Iγ1-Cμ) and post-recombination (Iμ-Cγ1) transcripts ( Fig. 7c ). 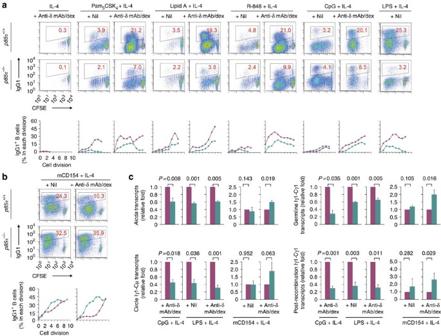Figure 7: BCR and TLR-induced CSR is impaired inp85α–/–B cells. (a) Proportions of sIgG1+B cells after stimulation of CFSE-labelled sIgδ+p85α–/–B cells (teal) and theirp85α+/+counterparts (plum) with Pam3CSK4(100 ng ml−1), lipid A (1 μg ml−1), R-848 (30 ng ml−1) or CpG (1 μM) in the absence or presence of anti-δ mAb/dex (100 ng ml−1), LPS (3 μg ml−1), all in the presence of IL-4 (3 ng ml−1), (top panels), and proportions of B cells at each cell division that were sIgG1+(bottom panels). (b) Proportions of sIgG1+B cells after stimulation of CFSE-labelled sIgδ+p85α–/–B cells (teal) and theirp85α+/+counterparts (plum) with mCD154 (1 U ml−1) plus IL-4 (3 ng ml−1), in the absence or presence of anti-δ mAb/dex (top panels), and proportions of B cells at each cell division that were IgG1+(bottom panels). (c) Levels ofAicda,germline Iγ1-Cγ1, circle Iγ1-Cμ and post-recombination Iμ-Cγ1 transcripts inp85α–/–B cells (teal) and theirp85α+/+counterparts (plum) stimulated with CpG (1 μM) and anti-δ mAb/dex (100 ng ml−1), LPS (3 μg ml−1) or mCD154 (1 U ml−1) in the absence of presence of anti-δ mAb/dex, plus IL-4 (3 ng ml−1). Data were normalized to the level ofCd79band are depicted as the ratio to the expression levels inp85α+/+B cells (mean and s.e.m. of data from three independent experiments;Pvalues:t-test). Figure 7: BCR and TLR-induced CSR is impaired in p85α –/– B cells. ( a ) Proportions of sIgG1 + B cells after stimulation of CFSE-labelled sIgδ + p85α –/– B cells (teal) and their p85α +/+ counterparts (plum) with Pam 3 CSK 4 (100 ng ml −1 ), lipid A (1 μg ml −1 ), R-848 (30 ng ml −1 ) or CpG (1 μ M ) in the absence or presence of anti-δ mAb/dex (100 ng ml −1 ), LPS (3 μg ml −1 ), all in the presence of IL-4 (3 ng ml −1 ), (top panels), and proportions of B cells at each cell division that were sIgG1 + (bottom panels). ( b ) Proportions of sIgG1 + B cells after stimulation of CFSE-labelled sIgδ + p85α –/– B cells (teal) and their p85α +/+ counterparts (plum) with mCD154 (1 U ml −1 ) plus IL-4 (3 ng ml −1 ), in the absence or presence of anti-δ mAb/dex (top panels), and proportions of B cells at each cell division that were IgG1 + (bottom panels). ( c ) Levels of Aicda, germline Iγ1-Cγ1, circle Iγ1-Cμ and post-recombination Iμ-Cγ1 transcripts in p85α –/– B cells (teal) and their p85α +/+ counterparts (plum) stimulated with CpG (1 μ M ) and anti-δ mAb/dex (100 ng ml −1 ), LPS (3 μg ml −1 ) or mCD154 (1 U ml −1 ) in the absence of presence of anti-δ mAb/dex, plus IL-4 (3 ng ml −1 ). Data were normalized to the level of Cd79b and are depicted as the ratio to the expression levels in p85α +/+ B cells (mean and s.e.m. of data from three independent experiments; P values: t -test). Full size image We further analysed the role of p85α-mediated BCR-signalling in activating the non-canonical NF-κB pathway. In p85α –/– B cells, in which BCR-signalling was defective whereas TLR- and CD40-signalling were intact, anti-δ mAb/dex- or LPS-induced p100 expression and processing to p52 were virtually abolished, but lipid A or CpG-induced p100 expression was normal, as was mCD154-induced p100 expression and processing to p52 ( Fig. 6b ; Supplementary Fig. S7b ). In addition, in these B cells, anti-δ mAb/dex enhancement of lipid A- or CpG-induced (canonical NF-κB) p65 phosphorylation was impaired, as was LPS-induced p65 phosphorylation ( Fig. 5 ; Supplementary Fig. S6b ); CpG- or mCD154-induced p65 phosphorylation, however, was largely unaffected. Thus, through PI(3)K, BCR-signalling activates the non-canonical NF-κB pathway and enhances the TLR-dependent canonical NF-κB pathway, thereby synergizing with TLRs in inducing AID and CSR. BCR/TLR-engaging NP–LPS induces switched NP-specific IgGs We next extended our in vitro findings to show that dual BCR/TLR engagement induces efficient CSR in vivo by injecting normal C57BL/6 mice with NP–LPS conjugate. This avoids proteinic linkages (such as in streptavidin used for conjugation to biotinylated moieties) that would introduce a T-cell-dependent component in the antibody response, thereby complicating the interpretation of results. The NP–LPS conjugate would also maximize the number of B cells hit with concomitant (NP-specific) BCR-crosslinking and TLR4-engagement, as the frequency of B cells expressing NP-specific BCR in the normal mouse B cell repertoire is only ~10 –7 (in our in vitro cultures, virtually all B cells were BCR-crosslinked by anti-δ mAb/dex). The presence of a large proportion of B cells expressing BCRs binding to the LPS polysaccharidic moiety was irrelevant, because such BCRs do not cross-react with NP. As predicted, NP–LPS induced a strong class-switched (IgG3 and IgG2b, and to a lesser extent IgG1 and IgG2a) NP-specific antibody response, which was readily detectable 6 days after injection and sustained through day 12 ( Supplementary Fig. S9 ). By contrast, a comparable class-switched NP-specific antibody response was not elicited by NP 26 (which efficiently crosslinks NP-specific BCRs but does not engage TLRs), or LPS alone. NP-binding to IgMs were detectable not only in mice injected with NP–LPS, but also and, to a lesser extent, in mice injected with NP 26 , likely owing to the decavalency and high avidity of this Ig class. Thus, these experiments show that, as predicted by our in vitro findings, dual BCR/TLR engagement in vivo induces class-switched and specific antibodies. The IgG subclasses (IgG3 and IgG2b) elicited by NP–LPS reflect those characteristically induced by LPS [6] . Here we have shown that BCR-signalling synergized with TLR1/2-, TLR4-, TLR7- or TLR9-signalling to induce AID and enable CSR. Either signalling alone resulted in marginal (TLRs) or no (BCR) CSR. Importantly, BCR crosslinking synergized with all TLR ligands analysed for CSR induction, thereby emphasizing the critical role of dual BCR/TLR-signalling in inducing specific and isotype-diverse antibodies at early stages of the response to bacteria or viruses, before T-cell help becomes available [3] , [4] . In addition, as emphasized by our in vivo demonstration that NP–LPS conjugate elicited a strong NP-specific IgG3 and IgG2b response, CSR induced by dual BCR/TLR engagement underpins the generation of class-switched Abs throughout T-independent responses, such as those involving bacterial or viral BCR-crosslinking antigens, together with TLR-engaging microbe-associated molecular patterns, such as LPS, Pam 3 CSK 4 , single-stranded RNA, polymerized flagellin, double-stranded RNA or unmethylated microbial DNA. The important role of B-cell TLRs in antibody responses to microbial pathogens is emphasized by reduced IgGs, particularly against pyogenic bacteria, in patients with defective TLR-signalling pathways [21] and decreased IgGs to protein antigens admixed with TLR ligands in TLR-, MyD88- and/or TRIF-deficient mice [3] , [4] . BCR and TLR synergy in inducing AID and CSR reflects the activation by these two receptors of the non-canonical and canonical NF-κB pathways. As we showed here, TLR ligands activated NF-κB in B cells only through the canonical pathway [2] . This was potentiated by BCR crosslinking [30] (particularly by anti-δ mAb/dex, which initiates sustained BCR-signalling [18] , [42] ), which also activated the non-canonical NF-κB pathway. BCR and TLRs reciprocally enhanced the main NF-κB pathway activated by the other receptor; integration of the two signalling pathways would occur at the level of p100 induction (non-canonical) and TRAF6 activation (canonical), leading to induction of p52 and p65, respectively ( Fig. 8 ). NF-κB p52 and p65 subunits, which are also induced by CD154 and, as we showed here, LPS, bind to the AICDA / Aicda promoter and enhancer elements, respectively, to upregulate AID gene expression. 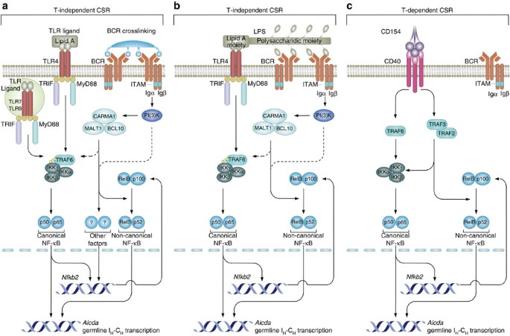Figure 8: BCR and TLR signalling are integrated to induce T-cell-independent CSR through both NF-κB pathways. (a) BCR crosslinking activates the non-canonical NF-κB pathway by inducing expression of p100 and its processing to p52 in a PI(3)K-dependent fashion. TLR engagement (as exemplified by TLR4 engagement by lipid A) activates the canonical NF-κB pathway, resulting in limitedAicdaexpression and marginal CSR. BCR enhances the TLR-dependent canonical NF-κB pathway, likely through TRAF6 activation, and TLR enhances the BCR-activated non-canonical NF-κB pathway by inducing p100 expression, thereby synergizing in inducing AID and CSR. (b) Unlike lipid A, LPS triggers both BCR-signalling through its polysaccharidic moiety and TLR4-signalling through its lipid A moiety, thereby activating both the non-canonical and canonical NF-κB pathways to induce AID and CSR in a PI(3)K-dependent fashion. (c) CD40 activation of the non-canonical and canonical NF-κB pathways and induction of CSR depend on TRAF2/TRAF3, which, however, play no role in the BCR-signalling pathway; TRAF6 mediates activation of the canonical NF-κB pathway only and is dispensable for CSR induced by CD40-signalling. Figure 8: BCR and TLR signalling are integrated to induce T-cell-independent CSR through both NF-κB pathways. ( a ) BCR crosslinking activates the non-canonical NF-κB pathway by inducing expression of p100 and its processing to p52 in a PI(3)K-dependent fashion. TLR engagement (as exemplified by TLR4 engagement by lipid A) activates the canonical NF-κB pathway, resulting in limited Aicda expression and marginal CSR. BCR enhances the TLR-dependent canonical NF-κB pathway, likely through TRAF6 activation, and TLR enhances the BCR-activated non-canonical NF-κB pathway by inducing p100 expression, thereby synergizing in inducing AID and CSR. ( b ) Unlike lipid A, LPS triggers both BCR-signalling through its polysaccharidic moiety and TLR4-signalling through its lipid A moiety, thereby activating both the non-canonical and canonical NF-κB pathways to induce AID and CSR in a PI(3)K-dependent fashion. ( c ) CD40 activation of the non-canonical and canonical NF-κB pathways and induction of CSR depend on TRAF2/TRAF3, which, however, play no role in the BCR-signalling pathway; TRAF6 mediates activation of the canonical NF-κB pathway only and is dispensable for CSR induced by CD40-signalling. Full size image Impairment of BCR-signalling, as in p85α –/– B cells, virtually abolished the generation of p52 following stimulation with anti-δ mAb/dex or LPS, thereby decreasing AID expression and CSR. This, together with the largely normal phosphorylation of p65 (despite a slight decrease in IκBα phosphorylation) in p85α –/– B cells and virtually no difference in proliferation and (limited) CSR between p85α –/– and p85α +/+ B cells on stimulation by CpG plus IL-4, strongly suggests that PI(3)K-signalling is more important for transducing BCR-signalling, than TLR-signalling, in B cells. The same time-dependence of p52 and AID induction, both of which progressively increased within 48 h and were perhaps linked to cell divisions, further emphasizes the critical role of the non-canonical NF-κB pathway in AID and CSR induction. Accordingly, unlike anti-δ mAb/dex, soluble/monomeric anti-Ig Abs cannot extensively crosslink BCR to initiate sustained signalling for activation of the non-canonical NF-κB pathway [43] or enhancement of AID and CSR [44] , [45] . Finally, BCR signalling, while upregulating AID and CSR and PNA-binding glycoproteins, downregulated Blimp1 and CD138, suggesting that antigen engagement of BCR delays plasmacytoid differentiation of TLR-stimulated B cells until CSR completion. We showed that BCR and TLRs synergized to induce CSR by enhancing AID expression rather than by merely promoting B-cell proliferation or survival. We also showed that BCR-enhanced and IL-4-dependent germline Iγ1-Cγ1 transcription peaked earlier than Aicda expression, thereby suggesting a synergy of the (BCR-activated) non-canonical NF-κB pathway, with the (IL-4R-activated) JAK-Stat6 pathway, to induce rapid gene expression. BCR enhancement of cytokine (IL-4, IFNγ and/or TGFβ)-promoted germline I H -C H transcription and TLR-dependent AID induction would underpin T-cell-independent CSR induction. Also, anti-δ mAb/dex, together with LPS, which induced B cells to undergo CSR to IgG3, induced high levels of post-translational modifications of histones in the Sγ3 DNA region [46] ; modified histones would stabilize 14-3-3 binding to S regions to unfold CSR [8] . The requirement for dual BCR/TLR engagement to induce efficient CSR can be fully satisfied by LPS alone. As we have shown, LPS, but not lipid A, induced CD79a phosphorylation (a unique hallmark of signalling emanating from BCR, but not from other receptors) and Ca 2+ mobilization, and activated the non-canonical NF-κB pathway, indicating that the LPS polysaccharidic moiety triggers BCR-signalling, which synergizes with lipid A moiety-engaged TLR4-signalling to induce AID expression and CSR. Indeed, blocking CD79a or deficiency in PI(3)K p85α hampered induction of CSR by LPS in the same fashion as it hampered induction of CSR by TLR ligands plus anti-δ mAb/dex. Findings that mice deficient in PI(3)K display negligible serum IgG3 and that B cells deficient in BCR-signalling elements, such as CD19, Btk, Blnk, Lyn or Vav, show greatly reduced responses to LPS [47] , [48] , [49] , [50] , [51] further support our conclusion that LPS activates BCR-signalling in addition to TLR4-signalling for CSR. The ability of O-antigen to bind (specific) BCRs to induce antibody responses to LPS in vivo [19] also provides strong support for the argument that the LPS polysaccharidic moiety engages the BCR and synergizes with the lipid A-engaged TLR4 to induce efficient CSR; polysaccharides have not been reported to interact with receptors on B cells other than the BCR [35] . Like dual BCR/TLR-signalling, including that triggered by LPS, CD40-signalling activates the two (non-canonical and canonical) NF-κB pathways for AID induction, demonstrating that T-cell-independent and T-cell-dependent CSR, despite their significant difference in the nature of triggering stimuli, entail the same set of transcription factors critical for AID induction ( Fig. 8 ). CD40, however, employs different signal transducers, utilizing TRAFs (TRAF2/TRAF3, in particular) to activate both NF-κB pathways and induce AID and CSR [52] —TRAF2 and TRAF3 have no role in the BCR-signalling pathway, thereby explaining the lack of synergy of BCR and CD40 in CSR. That CD40 activation of NF-κB and induction of AID and CSR were not impaired in p85α –/– B cells is also consistent with findings that BCR/PI(3)K-signalling has no significant role, or possibly even a negative role through Akt-mediated phosphorylation and, therefore, nuclear exclusion of Foxo1 (a transcription factor shown to enhance Aicda expression in CD40-dependent CSR [53] ); BCR-signalling, however, is required for CD40-dependent SHM [54] . BCR-triggered and time-dependent activation of the non-canonical NF-κB pathway versus nuclear exclusion of Foxo1 might influence the outcome of CD40-dependent CSR. Also, consistent with the dependence of IgA switching on TACI, which activates the canonical NF-κB pathway [55] , anti-δ mAb/dex synergized with TACI ligand BAFF or APRIL to induce CSR to IgA (our findings and ref. 28 ). Our findings that dual BCR/TLR engagement induced CSR in, up to, 40% of B cells indicate that T-cell-independent CSR can be as efficient as CD40-dependent CSR, as induced by specific CD4 + T-helper cells. They also provide much needed evidence for the argument that dual BCR/TLR engagement is highly relevant to T-independent antibody responses, a notion further supported by our in vivo experiments showing a strong NP-specific IgG response induced by NP–LPS, which is devoid of any proteinic component and, therefore, would not elicit T-cell help. In spite of (conflicting) suggestions on the ability of NP 26 (NP-Ficoll) to induce modest levels of class-switched antibodies (for example, refs 56 , 57 ), our experiments have clearly shown that NP 26 could not induce an in vivo class-switched NP-specific antibody response comparable to that induced by NP–LPS, further extending our in vitro findings that BCR crosslinking alone did not efficiently induce AID or CSR. Collectively, our in vitro and in vivo findings indicate that among the pool of B cells that can be activated by TLR ligands, only those that can also bind to antigen can undergo TLR-dependent differentiation, thereby focusing the early adaptive (antibody) response when specific T-cell help is not yet available or effectively mediating antibody response to some T-independent antigens. They outline a major T-independent B-cell differentiation pathway, as underpinned by dual BCR/TLR induction of AID and CSR, to diversify antibody responses. Such a pathway would be evolutionarily conserved in jawed vertebrates, which express germline encoded and nonclonally distributed TLRs and clonally distributed BCRs. In organisms with a primitive adaptive immune system, for example, jawless vertebrates, cooperation of TLRs or perhaps other innate immune receptors with antigen receptor VLRB [58] might have an important role in fighting invading pathogens. B cells Single B-cell suspensions were prepared from murine axillary, inguinal and cervical lymph nodes using a 70-μm cell strainer. Spleen B cells were resuspended in ACK Lysis Buffer (Lonza) to lyse red blood cells, quenched with RPMI containing 10% FBS (RPMI-FBS) and then resuspended in same medium before further B-cell purification. Lymph node and spleen B cells were purified by negative depletion of cells expressing CD43, CD4 or Ter-119 using the B cell Isolation kit (Miltenyi), following manufacturer's protocol, resulting in a preparation of more than 99% B220 + sIgδ + B cells ( Supplementary Fig. S10 ). In most experiments, we supplemented the kit with biotinylated mAb to CD11c (clone N418, eBioscience) and mAb to IgG1 (clone A85-1, BD Biosciences), thereby achieving an even greater degree of sIgδ + B cell purity. B-cell-surface analysis and proliferation sIgδ + B cells were stimulated for 4 days and collected for flow cytometry analysis of surface expression of Ig, B220, CD138 or PNA-binding glycoproteins ( Supplementary Table S1 ), as we had described [8] , [11] . For proliferation studies, B cells were resuspended in PBS at 10 7 cells per ml and incubated with 4 μ M of carboxyfluorescein diacetate succinimidyl ester (Invitrogen) at 37°C for 5 minutes and immediately quenched with 10 vol of RPMI-FBS. Cells were analysed using a BD FACSCalibur (BD Biosciences) and data analysis was performed using the FlowJo software (Tree Star). Dead cells (7–AAD + ) were excluded from analysis. Cell divisions were determined using the proliferation platform of FlowJo. CSR sIgδ + B cells were cultured at 10 5 cell ml −1 in RPMI–FBS supplemented with 50 μ M β-mercaptoethanol in the presence of the following stimuli at the indicated dose, unless otherwise specified: TLR1/2 ligand Pam 3 CSK 4 (100 ng ml −1 , Invivogen), TLR4 ligand monophophoryl lipid A (lipid A, 1 μg ml −1 , Sigma-Aldrich), TLR7 ligand R-848 (30 ng ml −1 , Invivogen) or TLR9 ligand CpG ODN1826 with a phosphorothioate backbone (CpG, 1 μ M , sequence 5′-TCCATGACGTTCCTGACGTT-3′; the sequence of the control GpC ODN 1745 was 5′-TCCATGAGCTTCCTGAGTCT-3′; Operon), LPS deproteinized by chloroform extraction (3 μg ml −1 , from E. coli , serotype 055:B5, Sigma-Aldrich), mCD154 (1 U ml −1 ), BAFF (250 ng ml −1 , Alexis) or APRIL (250 ng ml −1 , Alexis). mCD154 was obtained by expression of mouse CD154 on membranes of Sf21 insect cells [8] . Rat anti-mouse δ chain mAb (clone 11-26)-conjugated to dextran [18] (anti-δ mAb/dex, Fina Biosolutions) was added where indicated. Recombinant IL-4 (3 ng ml −1 ) was added for CSR to IgG1 and IgE; IFNγ (25 ng ml −1 ) for CSR to IgG2a and IgG3 where indicated; IL-4 (3 ng ml −1 ), IL-5 (3 ng ml −1 ) and TGFβ (2 ng ml −1 ) for CSR to IgA (cytokines were all from R&D Systems). Real-time qRT–PCR transcript analysis RNA was extracted from 5×10 6 B cells stimulated for 48 h (or as indicated) using the RNeasy Mini Kit (Qiagen). First-strand complementary DNA was synthesized from equal amounts of total RNA (4 μg) using the SuperScript III System (Invitrogen) and analysed by the SYBR Green dye (Bio-Rad) incorporation in PCR reactions involving specific primers ( Supplementary Table S2 ) and performed in an iCycler and MyIQ real-time qPCR system (Bio-Rad). The levels of transcripts were quantified by the ΔΔCT (cycle threshold) method. Ca 2+ mobilization assay For analysis of the elevation of [Ca 2+ ] cytosol induced by transient BCR-signalling, B cells were loaded with Fluo-3 AM (5 μg ml −1 , Invitrogen) and Fura-Red AM (10 μg ml −1 ) in 1 ml of RPMI containing 2% (v/v) of FBS and 0.04% (v/v) of pluronic F-127 at 37°C for 45 m. After washing with HBSS containing 1% (g/v) of BSA, 1 m M of CaCl 2 and 1 m M of MgCl 2 (HBSS-Ca), cells were pelleted and resuspended in 500 μl of HBSS-Ca and stained with APC-conjugated anti-B220 mAb (eBiosciences). After washing, cells were resuspended in HBSS-Ca, stimulated with F(ab′)2 of goat anti-mouse μ chain (anti-μ F(ab′)2, Southern Biotech) or anti-δ mAb/dex at indicated concentrations and immediately analysed by flow cytometry. The level of free intracellular Ca 2+ was determined by the ratio of the Fluo-3 intensity to the Fura-Red intensity using the 'kinetics' tool of the FlowJo software. For analysis of Ca 2+ mobilization following a long period of stimulation, resting B cells were stimulated for 16 h with anti-δ mAb/dex or LPS, or nil, lipid A or mCD154 and labelled with Fluo-3 AM and Fura-Red as above, and then stimulated with anti-μ F(ab′) 2 (5 μg ml −1 ) and analysed. CD79a phosphorylation assay Spleen B cells (10 7 ) were stimulated as indicated, collected and resuspended in lysis buffer (20 m M of Tris–Cl, pH 7.5, 150 m M of NaCl, 0.5 m M of EDTA, 1% (v/v) of NP-40) supplemented with phosphatase inhibitors sodium pyrophosphate (1 m M ), NaF (10 m M ) and NaVO 3 (1 m M ) and a cocktail of protease inhibitors (Sigma). After sonication and centrifugation, protein lysates were pre-cleared with protein A-agarose (Pierce) for 2 h at 4°C and then incubated with Armenian hamster anti-mouse CD79a (2 μg ml −1 , BioLegend) or control IgGs with irrelevant specificities overnight at 4°C before immunocomplexes were precipitated by protein A-agarose beads. After washing with lysis buffer, proteins were eluted in SDS sample loading buffer and separated by SDS–PAGE. After transferring onto nitrocellulose membranes, proteins were subjected to immunoblotting involving anti-phosphoCD79a(Tyr182) Ab (Cell Signaling Technology). NF-κB activation assays Spleen B cells (10 7 ) were resuspended in RPMI-FBS and stimulated as indicated. Cell lysates were separated by SDS–PAGE and transferred onto nitrocellulose membranes. Membranes were subjected to sequential immunoblotting with anti-phosphoIκBα or anti-phosphop65 mAb (Cell Signaling Technology; the canonical NF-κB pathway) or anti-p52 Ab (also detecting p100, Santa Cruz; the non-canonical NF-κB pathway). For analysis of the non-canonical NF-κB pathway, membranes were stripped in 200 m M of glycine (pH 2.5) at 25 °C for 1 h and subjected to immunoblotting involving anti-β-actin mAb (Sigma-Aldrich). For analysis of the canonical NF-κB pathway, membranes were stripped and subjected to immunoblotting involving anti-IκBα or anti-p65 mAb, and stripped again for immunoblotting involving anti-β-actin mAb. Signals were quantified using the ImageJ software (NIH). Retroviral transduction The Aicda coding sequence was cloned into the retroviral vector pCSretTAC (pTAC, as we described [11] ), which contains the human IL2RA coding sequence (encoding the TAC antigen, CD25), to generate the pTAC–AID retroviral vector. Generation of retroviruses in HEK-293 T cells was as we described [11] . For transduction and CSR analysis, mouse B cells were activated by CpG in the absence or presence of anti-δ mAb/dex plus IL-4 for 24 h and then incubated with virus in the presence of 6 μg ml −1 polybrene (Sigma-Aldrich) for 90 m. After culture media were replaced with virus-free media, cells were cultured with CpG or anti-δ mAb/dex plus IL-4 for 72 h for sIgG1 expression analysis, or for 48 h for transcript analysis, as we described [8] , [11] . Mice and immunization C57BL/6 mice deficient in p85α ( p85α –/– ) were generated after backcrossing of previously described p85α –/– mice in the Balb/c genetic background [59] onto the C57BL/6 background for 9 generations (Taconic). In these mice, mature lymph node B cells were virtually normal in development despite defective development of spleen marginal zone B cells [38] , [59] . Mice used in all experiments were 8–12 weeks of age and without any apparent infection or disease, and were housed in a pathogen-free animal vivarium facility at UC Irvine. All protocols were in accordance to the regulations of the UC Irvine IACUC. C57BL/6 mice were injected intraperitoneally with 4-hydroxy-3-nitrophenylacetyl (NP) conjugated to LPS (NP–LPS) (average: 0.2 NP molecule conjugated with one LPS molecule; Biosearch; 25 μg), NP 26 (average: 26 NP molecules immobilized on one Ficoll molecule; Biosearch; 25 μg) or LPS (25 μg), all in PBS (100 μl) without adjuvant and sera were collected before injection and 6 days and 12 days after injection. Total and NP-specific antibody concentrations Total IgM, IgG1, IgG2a, IgG3, IgA and IgE concentrations in supernatants from B-cell cultures or NP-specific IgM, IgG1, IgG2a, IgG2b and IgG3 concentrations in sera of immunized mice were determined by specific ELISAs as we reported previously [8] , [11] . Statistical analysis Statistic analysis was performed by either GraphPad (Prism) or Excel (Microsoft) software to determine P values by paired student t -test. How to cite this article: Pone, E.J. et al . BCR-signalling synergizes with TLR-signalling for induction of AID and immunoglobulin class-switching through the non-canonical NF-κB pathway. Nat. Commun. 3:767 doi: 10.1038/ncomms1769 (2012).